Tumour lineage-homing cell-penetrating peptides as anticancer molecular delivery systems Cell-penetrating peptides have gained attention owing to their promise in noninvasive delivery systems. Among the identified cell-penetrating peptides, the TAT peptide has been preferentially used for transduction into cells of diverse origins. However, this activity is nonselective between neoplastic and non-neoplastic cells. Here we describe artificial cell-penetrating peptides that are selectively and efficiently incorporated into human tumour cells, according to their lineage. Ten representative tumour lineage-homing cell-penetrating peptides were obtained by screening of a random peptide library constructed using messenger RNA display technology, and some of the isolates were further modified by amino-acid substitution. Their advantageous tumour cell-targeting ability is corroborated in an in vivo mouse model for imaging and growth suppression of metastatic xenoplant tumours. These cell-penetrating peptides are potentially useful for the efficient targeting of human neoplasms in a tumour origin-dependent manner, and provide a framework for the development of peptide-based anti-tumour technologies. Partial amino-acid sequences encoded by several viral and cellular proteins have recently been found to penetrate cells via the surface plasma membrane [1] . These distinctive peptides, termed 'cell-penetrating peptides', or CCPs, (also called PTDs; protein transduction domains), have a role in noninvasive, minimally cytotoxic transport via physiological mechanisms such as macropinocytosis and endocytosis [13] . Accordingly, CPP sequences have been used to generate CPP-molecular fusions, leading to the development of cell-permeable peptide/proteins, nucleic acids, and small chemical compounds, as well as imaging probes for diagnostics. TAT peptide, which is a CPP, has been heavily utilized for its high solubility and diverse target range, although its nonselective internalization is a limiting factor for specific cell-targeting applications [13] . Random peptide libraries constructed by messenger RNA display technology are more tailored for isolating CPPs than phage display, as the former are comprised of RNA/cDNA-peptide chimeric molecules lacking any phage components [13] . Consequently, the molecular size of an mRNA display-based complex is considerably smaller than a phage displayed peptide. Moreover, the number of peptides displayed is larger, which increases the efficiency of the screen. Here we applied mRNA display technology to obtain novel CPPs as tumour lineage-homing CPPs. We found that it was possible to target specific tumour cell types with different CPPs and discuss their potential for peptide-based molecule delivery systems. Isolation of tumour lineage-homing CPPs Jurkat, CHO, or HeLa cells were incubated in medium with the mRNA display library solutions containing puromycin-anchored randomized mRNA/cDNA-peptide chimeras for 1 h each. Cells from each sample were subsequently collected and the extracted cDNAs were amplified by PCR. We then sequentially reconstituted the library as previously described [7] ( Fig. 1a ). Repeating this cycle five to six times, amino-acid sequences were identified as primary candidates for CPPs. Fluorescein isothiocyanate (FITC)-conjugated forms of these novel 15 amino-acid-long CPPs were subjected to further analysis, which included amino-acid-substituted derivatives [7] generated from sequence information of intracellularly incorporated molecules. During the first screen to examine the cell permeability of these peptides using Jurkat, CHO and HeLa cells, we found that several of them showed a distinct cell type-dependent penetrative activity. On the basis of this finding, by screening of 47 synthesized peptides, we attempted to identify CPPs with unique permeability across human neoplastic cells, using a broad range of malignant tumour lines of different cellular origins ( Fig. 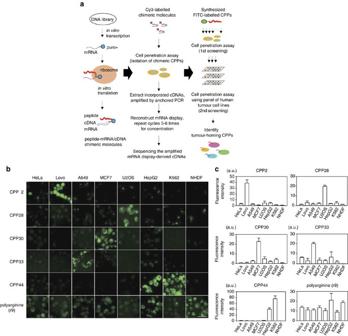Figure 1: Isolation of tumour-lineage homing cell-penetrating peptides. (a) Construction of mRNA display-molecules and outline of screening method for isolation of tumour-homing CPPs. The library was constructed as previously described7. (b) Five representative tumour lineage-homing CPPs that showed selective permeation obtained from the assay. Fluorescence images of tumour cell lines by cell penetration assay are shown according to each numbered CPP. CPP2, colon cancer lineage-homing; CPP28, osteosarcoma-homing; CPP30, breast cancer-homing; CPP33, lung adenocarcinoma-homing; CPP44, highly selective permeation both to hepatocellular carcinoma and leukaemia. Nona-arginine (polyarginine; r9) was employed as a representative for nonselectively permeable CPP. Scale bar, 10 μm. (c) Quantitative analysis of selective permeability of each tumour lineage-homing CPP among eight cell lines with different origins. Relative fluorescence intensity of individual cells against background was calculated in each image obtained by fluorescence microscopy as shown in (c). a.u., arbitrary unit. Means and s.d. of triplicates are shown. 1a ; Table 1 ). Normal human dermal fibroblasts (NHDF) were included as a non-neoplastic counterpart. Briefly, 10 μM of each FITC-labelled peptide were incubated with each cell line for 6 h, followed by thorough washing out of extracellular peptides, after which living cells were examined by inverted fluorescence microscopy. 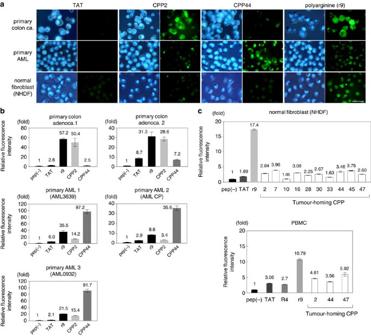Figure 2: Penetrating efficiency of tumour lineage-homing CPPs to target tumour cells. (a) Primary tumour cells were prepared from surgically excised or biopsied patient tissues. Neither CPP was significantly incorporated into NHDF in comparison with each tumour. All indicated peptides were used at 10 μM. Scale bar, 10 μm. (b) FACS quantification of fluorescence intensity for individual primary tumour lines treated with the indicated CPPs. 10 μM of each CPP was introduced, the extracellular peptide was thoroughly washed out, and living samples were analysed after a 3-h incubation. Columns represent the mean fluorescence intensity of each sample relative to the intensity of the untreated cells (1.0). Means and s.d. of triplicates are shown. (c) Incorporation of tumour-homing CPPs to non-neoplastic cells. Intracellular uptake of the indicated CPPs to NHDF and PBMC were quantified by FACS. CPP16 seq.: RLWMAWYSPTTRRYG. Means and s.d. of triplicates are shown. This method identified ten CPPs that uniquely permeated tumour cells differing in their lineage backgrounds ( Table 2 ). Fluorescent cellular images were taken for demonstrating these penetrating activities ( Supplementary Fig. S1a ). Five of the initial ten CPPs are shown as representative tumour-homing CPPs compared with polyarginine (r9) [8] , which nonselectively penetrates all neoplastic and non-neoplastic cells ( Fig. 1b ). For example, CPP2 showed highly efficient permeation of the colon adenocarcinoma cell line, Lovo, without any significant uptake by the other tumour cell lines. CPP7 was observed to be highly permeable in H28 cells (malignant mesothelioma), CPP28 in U2OS cells (osteosarcoma), CPP30 in MCF-7 cells (breast carcinoma), and CPP33 in A549 cells (lung adenocarcinoma), indicating tumour-lineage selective penetration ( Fig. 1b ; Supplementary Fig. S1a ). In the case of CPP44, elevated transduction took place in both myelogenous leukaemia K562 and hepatoblastoma HepG2. Despite being readily incorporated into tumour cells, CPP44 incorporation was restricted to a very limited range of tumours ( Fig. 1b ). In contrast to these, both CPP10 and CPP45 transduced a broad range of solid tumour cells covering both carcinomas and sarcomas, although the transduction efficiency fluctuated depending on the tumour line ( Supplementary Fig. S1a ). The efficiency of intracellular incorporation of each CPP was quantitatively measured by detecting the fluorescence intensities of individual living cells in the tumour lines treated with the peptides ( Fig. 1c ; Supplementary Fig. S1b ). CPP47 and CPP48, which permeated solid tumours poorly, penetrated haematopoietic malignancies including leukaemias and lymphomas ( Supplementary Fig. S1c ). All of these CPPs showed poor incorporation into normal human fibroblasts, NHDF, with the same dose. Figure 1: Isolation of tumour-lineage homing cell-penetrating peptides. ( a ) Construction of mRNA display-molecules and outline of screening method for isolation of tumour-homing CPPs. The library was constructed as previously described [7] . ( b ) Five representative tumour lineage-homing CPPs that showed selective permeation obtained from the assay. Fluorescence images of tumour cell lines by cell penetration assay are shown according to each numbered CPP. CPP2, colon cancer lineage-homing; CPP28, osteosarcoma-homing; CPP30, breast cancer-homing; CPP33, lung adenocarcinoma-homing; CPP44, highly selective permeation both to hepatocellular carcinoma and leukaemia. Nona-arginine (polyarginine; r9) was employed as a representative for nonselectively permeable CPP. Scale bar, 10 μm. ( c ) Quantitative analysis of selective permeability of each tumour lineage-homing CPP among eight cell lines with different origins. Relative fluorescence intensity of individual cells against background was calculated in each image obtained by fluorescence microscopy as shown in ( c ). a.u., arbitrary unit. Means and s.d. of triplicates are shown. Full size image Table 1 List of human tumour cell lines for CPP screening. Full size table Table 2 Ten tumour lineage-homing cell penetrating peptides identified from the mRNA display library. Full size table Following these results, we further confirmed CPP selective permeability to tumour cell lineages using several different tumour lines of the same origin. For example, the strong permeation observed in Lovo by CPP2 was corroborated in three additional colon adenocarcinoma lines, Sw620, Colo320 and WiDr, whereas other lineages such as MCF-7 and NHDF ( Supplementary Fig. S2a ) again did not show significant permeation. Additionally, CPP44 penetrated five hepatic tumour lines, including the hepatoblastoma line, HepG2, and the hepatocellular carcinoma lines, KYN-1, KYN-3, HAK-1B [9] and HLE, but not two lines, Hep3B and Huh-7 ( Supplementary Fig. S2a ). Moreover, CPP44 could not only penetrate K562 cells, as shown in Fig. 1b , but also penetrated five cases of acute myelogenous leukaemias (AMLs) ( Supplementary Fig. S2a ). On the basis of these results, we focussed on the colon cancer-homing CPP2 and leukaemia-homing CPP44, as representative examples. We first examined whether the CPPs isolated from mRNA display libraries are able to target not only established cell lines, but also primary tumour cells directly isolated from cancer patients. CPP2 or CPP44 (both 10 μM) were incubated for 3 h with primary colon adenocarcinoma cells, primary AML cells, and normal fibroblasts, respectively ( Fig. 2a ). The same concentration of TAT and nona-D-arginine (r9) were employed as controls. In contrast to TAT and CPP44, CPP2 was successfully internalized by primary colon adenocarcinoma cells. Similarly, primary myelogenous leukaemic cells (AML) showed uptake of CPP44, but not of TAT or CPP2 at comparable concentrations. These three CPPs showed poor penetration into normal fibroblasts, whereas r9 was nonselectively incorporated into all tumour cells and fibroblasts. The efficiency of permeability into primary tumour cells was also evaluated in addition to their linage-homing characteristics, as was done for established tumour lines. Flow cytometric analysis revealed FITC-labelled CPP2 penetrated primary colon cancer cells 3- to 15-fold more efficiently than TAT or CPP44, although r9 showed a similar efficiency to CPP2 ( Fig. 2b ). CPP44 potently permeated primary AML tumour cells isolated from three different patients (termed AML3639, AML CP and AML0932), over tenfold more than TAT, fourfold more than r9, and six- to ten-fold more than CPP2 ( Fig. 2b ). Thus, CPP2 and CPP44 are expected to be applicable to primary colon cancer cells and AML cells from patients, respectively. Figure 2: Penetrating efficiency of tumour lineage-homing CPPs to target tumour cells. ( a ) Primary tumour cells were prepared from surgically excised or biopsied patient tissues. Neither CPP was significantly incorporated into NHDF in comparison with each tumour. All indicated peptides were used at 10 μM. Scale bar, 10 μm. ( b ) FACS quantification of fluorescence intensity for individual primary tumour lines treated with the indicated CPPs. 10 μM of each CPP was introduced, the extracellular peptide was thoroughly washed out, and living samples were analysed after a 3-h incubation. Columns represent the mean fluorescence intensity of each sample relative to the intensity of the untreated cells (1.0). Means and s.d. of triplicates are shown. ( c ) Incorporation of tumour-homing CPPs to non-neoplastic cells. Intracellular uptake of the indicated CPPs to NHDF and PBMC were quantified by FACS. CPP16 seq. : RLWMAWYSPTTRRYG. Means and s.d. of triplicates are shown. Full size image To examine the incorporation of the CPPs into non-neoplastic counterparts, NHDF and peripheral blood mononuclear cells (PBMC) were chosen as examples for cell-penetration assays with the same. Fluorescence-activated cell sorting (FACS) analysis showed r9 was the most potent peptide to permeate NHDF, whereas the permeability's of tumour-homing CPPs were considerably weaker, comparable to TAT ( Fig. 2c ). Similarly, TAT, tetra-L-arginine (R4), CPP2, CPP44, and CPP47 showed poor penetration in PBMC, although r9 was comparably permeant ( Fig. 2c ). As complete conversion of a CPP into its retro-inverse sequence has been reported to enhance permeability [8] , the permeability of the retro-inverse CPP44 (RI-CPP44; kmpnwtyrfmtprk) was examined against target cells. However, the retro-inverse form exhibited reduced permeation into primary AML cells ( Supplementary Fig. S2b ). Mechanism of internalization of tumour-homing CPPs Next, we investigated the molecular mechanism of the tumour lineage-homing permeability of these CPPs. To reveal the primary physiological pathway of incorporation, two representative CPPs, colon cancer-homing CPP2 and myeloid leukaemia-homing CPP44, were chosen as examples. First, their internalization was examined using 5-( N -ethyl- N -isopropyl) amiloride (EIPA) [10] , Dynamin inhibitor I (DI; Dynasore) [11] , and chlorpromazine (CPZ) [12] . Pretreatment of the cells with EIPA, a macropinocytosis inhibitor, prevented the entry of polyarginine (r9) [13] in a dose-dependent manner; however, the entry of CPP44 into primary AML cells was not impeded. CPP2 permeation into the colon cancer line Lovo was not impeded in the presence of EIPA either ( Fig. 3a ). Both CPPs failed to permeate at 4 °C, whereas the absence of serum did not impair penetration (data not shown). This indicates that these CPPs are ATP-dependently incorporated, and that the mechanism of uptake was not mediated by serum components. When the cells were pretreated with DI, neither CPP44 nor CPP2 penetrated in target cells ( Fig. 3b ). However, CPZ, an inhibitor of clathrin-dependent endocytosis, did not prevent cell entry ( Fig. 3c ). Uptake of FITC-labelled transferrin was inhibited by the same concentration of DI and CPZ ( Supplementary Fig. S2c ). These results indicate that cellular entry of CPP44 and CPP2 is mediated by a dynamin-dependent and clathrin-independent endocytic pathway [14] . We further investigated the molecular mechanism of CPP44 incorporation into myelogenous leukaemia cells using a short interfering RNA (siRNA) library to identify the critical genes for its uptake. Library screening of 1,905 siRNAs against human receptor genes revealed M160 (CD163L1) , macrophage/monocyte scavenger receptor cysteine-rich type 1 protein of the CD163 family [15] , to be a critical regulator of CPP44 incorporation into leukaemic cells. M160 mRNA knockdown by specific siRNA in AML cells significantly impaired intracellular uptake of CPP44 ( Fig. 3d ; Supplementary Fig. S2d ). The same phenomenon was also observed in HepG2 by knockdown of M160 mRNA ( Supplementary Fig. S2d ). A decrease of M160 affected incorporation, but did not seem to completely abrogate CPP44 uptake into these tumour cells, suggesting that additional genes may cooperate with M160 in the molecular mechanism. Although the function of M160 in a variety of malignant tumours still remains unclear, both M160 mRNA and protein are abundantly expressed in myelogenous leukaemia-lineage cells (K562, AML3639, AML CP, and AML0932) in contrast to other lineages of tumours ( Fig. 3e ). A similar tendency was also recognized in hepatic tumour lines. Lines with an elevated intracellular uptake of FITC-CPP44 express M160 at a higher level than lines lacking internalized peptide normal liver cells and fibroblasts do not show any M160 expression ( Supplementary Fig. S2e ). Moreover, CPP44 did not penetrate into non-neoplastic liver cells, while it preferentially permeated hepatic tumour lines ( Supplementary Fig. S2e ). Conversely, CPP48 permeated normal liver cells with significantly low permeability in hepatic tumour cell lines. 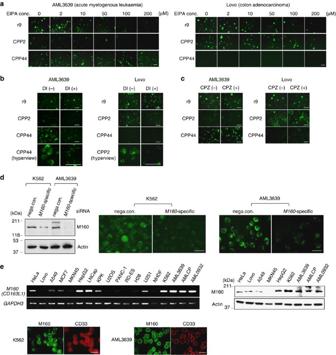Figure 3: Internalization mechanism of tumour lineage-homing CPP to target cells. (a) Effect of a macropinocytosis inhibitor, EIPA, on CPPs. Internalization of polyarginine (r9) was disturbed in a dose-dependent manner. The internalization of CPP44 into AML cells was not affected by EIPA. Similarly, uptake of CPP2 by the colon adenocarcima cell line Lovo was not affected by EIPA. 2 μM of each peptide was used. (b) Dynamin inhibitor I blocked penetration of Cpp2 and CPP44 into the target cells (DI; Dynasore, 80 μM, 1-h incubation). (c) Chlorpromazine, an inhibitor of clathrin-dependent endocytosis, did not affect the uptake of CPP2 and CPP44 (CPZ; 20 μM, 1-h incubation). (d) Knockdown ofM160by siRNA and its effect on myelogenous leukaemia cells. 50 nM of siRNAs againstM160were introduced. 2 μM of FITC-labelled CPP44 was evaluated 3 h post-transduction. (e) mRNA and protein expression ofM160on tumour cells with a different origin. Fluorescence images of M160 (FITC) and CD33 (cy3) in myelogenous leukaemia cells (K562 and AML3639). Scale bars (a,b,c,d,e), 10 μm. Figure 3: Internalization mechanism of tumour lineage-homing CPP to target cells. ( a ) Effect of a macropinocytosis inhibitor, EIPA, on CPPs. Internalization of polyarginine (r9) was disturbed in a dose-dependent manner. The internalization of CPP44 into AML cells was not affected by EIPA. Similarly, uptake of CPP2 by the colon adenocarcima cell line Lovo was not affected by EIPA. 2 μM of each peptide was used. ( b ) Dynamin inhibitor I blocked penetration of Cpp2 and CPP44 into the target cells (DI; Dynasore, 80 μM, 1-h incubation). ( c ) Chlorpromazine, an inhibitor of clathrin-dependent endocytosis, did not affect the uptake of CPP2 and CPP44 (CPZ; 20 μM, 1-h incubation). ( d ) Knockdown of M160 by siRNA and its effect on myelogenous leukaemia cells. 50 nM of siRNAs against M160 were introduced. 2 μM of FITC-labelled CPP44 was evaluated 3 h post-transduction. ( e ) mRNA and protein expression of M160 on tumour cells with a different origin. Fluorescence images of M160 (FITC) and CD33 (cy3) in myelogenous leukaemia cells (K562 and AML3639). Scale bars ( a , b , c , d , e ), 10 μm. Full size image According to its predicted secondary structure, CPP44 is comprised of a turn near the amino terminus and carboxy-terminal helical part followed by a beta-sheet structure. The penetrating activity of CPP44 into its target cells was maintained despite amino-acid substitutions at position 7 within the CPP44 peptide, where phenylalanine (F) was exchanged with either glutamine (E) or alanine (A), generating CPP44 F7E and CPP44 F7A peptides, respectively ( Supplementary Fig. S3a ). In contrast, permeability was impaired in response to phenylalanine replacement with proline (CPP44 F7P). On the basis of predicted structural information, CPP44 F7P loses the acute angled-winding structure, depicted by the green arrow, owing to the extension of the turn structure ( Supplementary Fig. S3b ). This may impede CPP44 binding to M160 at the cell surface. Growth suppression of primary tumour cells We next attempted to develop a tumour cell-selective molecular targeting system by taking advantage of these CPPs. Loss of p16 INK4a tumour expression is frequently observed in many biologically aggressive tumours [16] , [17] , [18] . The primary colon adenocarcinoma cells, from two patients, and primary AML cells, from three patients, shown in Fig. 2b were employed for a growth suppression assay examining both CPP2 and CPP44-fusion anti-tumour peptide. In all cases, p16 mRNA expression was absent ( Fig. 4a ), which is frequently observed in tumour cell lines of various origins ( Supplementary Fig. S4a ). Anti-tumour peptides were designed by fusing CPP44 or CPP2, as cell-penetrating domains, to the minimal inhibitory sequence of p16 (p16MIS) that has been reported to restore lost p16 function via GPG sequence [19] , [20] , [21] ( Fig. 4b ). We generated three different CPP44-fusion peptides for targeting primary leukaemic cells ( Fig. 4b ). CPP44-p16MIS was entirely comprised of L -polypeptide. By contrast, a retro-inverso sequence using D -amino acids was applied to the p16MIS motif in CPP44-RI-p16MIS, based on the finding that the retro-inverso form of the p16 MIS sequence augmented its binding affinity for the Cdk4/CyclinD1 complex by up to threefold compared with the original, according to BIACORE assay ( Fig. 4c ). The CPP44-RI-p16V95E peptide, a negative control that substitutes valine 95 (V95) in the MIS sequence with glutamate (E), showed minimal affinity to the target complex. CPP2-RI-p16MIS was prepared in the same manner for inhibiting colonic tumour growth. For all these anti-tumour peptides, four arginine residues were added to the C-terminus of each via GP-spacers to increase solubility. The CPP44-RI-p16MIS and CPP2-RI-p16MIS peptides successfully permeated into AML cells and colon adnocarcinoma cells, respectively, without compromising CPP target specificity ( Fig. 4d ). RI-p16MIS-4R, lacking the CPP44 sequence, did not penetrate into AML cells ( Fig. 4b, d ). The peptides were then introduced into endogenously p16-negative primary AML cells to monitor apoptosis induction by FACS analysis, using Annexin V. Leukaemic cells in all three cases of CPP44-RI-p16MIS treatment showed maximal cytocidal effects in a dose-dependent manner (~50% of the cells were apoptotic with 10 μM peptide at 24 h post-transduction) ( Fig. 5a ). As a transduction domain, CPP44 itself did not show cellular toxicity with the same dose. Replacement of the CPP44 sequence by TAT reduced apoptotic induction in primary AML cells by RI-p16 peptide from 58.4 to 23.8% at 20 μM 24 h post-introduction ( Supplementary Fig. S4b ). Moreover, CPP44-RI-p16MIS peptide did not significantly affect the viability of PBMC, which endogenously retains p16 expression, below 20 μM ( Supplementary Fig. S4c ). As 67% of the 10 μM CPP44-RI-p16MIS-treated cells became apoptotic at 48 h post-introduction, the cytocidal effect of the peptide seemed to be maintained at least for a few days by a single treatment ( Supplementary Fig. S4d ). Phosphorylated pRB protein levels time-dependently decreased in CPP44-RI-p16MIS-treated leukaemic cells ( Fig. 5b ), consistent with the induction of cell cycle arrest ( Supplementary Fig. S4e ), demonstrating that the peptide functioned in a target gene-specific manner as evidence of p16 restoration. Similarly, the CPP2-RI-p16MIS anti-tumour effect against primary colon cancer cells was also examined and it triggered apoptosis in a dose-dependent manner ( Fig. 5c ). When CPP2-RI-p16MIS was applied to AML cells, it triggered apoptosis in 22% of AML cells, which was less than its apoptotic efficiency (66%) in colon cancer cells ( Fig. 5d; Supplementary Fig. S4f ). In contrast, apoptosis triggered by CPP44-RI-p16MIS in colon cancer cells was one-fourth of that in leukaemic cells ( Fig. 5d ). Taken together, these data suggest that choosing the appropriate CPP will provide the most efficient anti-tumour outcomes for a particular lineage. For non-neoplastic cells such as NHDF, CPP44-RI-p16MIS did not significantly affect viability at doses effective for tumour cell suppression ( Fig. 5e ). CPP44-RI-p16MIS did not suppress the growth of a p16 -negative CML cell line, K562, despite its substantial peptide uptake, which was presumably because of a lack of pRB expression downstream of the p16/Cdk4/CyclinD1 pathway ( Fig. 5f ). 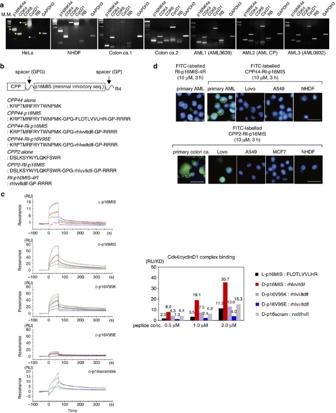Figure 4: Design of CPP-fusion anti-tumour peptide restoring p16INK4a function. (a) RT–PCR analysis of thep16tumour suppressor gene and its target gene expression in the indicated primary tumour cells. HeLa and NHDF; positive control. Arrowheads depict the PCR product of each gene. (b) Anti-tumour peptide design. Capital letters;L-amino acid. Lower case letters;D-amino acid. Each peptide was tagged with four arginines at its C-terminus to enhance solubility. (c) Specificity of the interaction of the retro-inverso-designed p16MIS peptide targeting p16, the Cdk4/CyclinD1complex. Real-time BIACORE sensorgrams of the interaction between the indicated peptide and the Cdk4/CyclinD1 protein complex, and the graph as a summary. Loaded peptide; 0.125, 0.25, 0.5, 1, 2 μM conc., respectively. RU; resonance unit, RU/KD; Relative Response/Molecular weight.D-p16MIS, the retro-inverso form of p16MIS showed maximum affinity to the target protein complex with the same doses. (d) Permeability of the CPP44- or CPP2-fusion chimeric p16MIS anti-tumour peptides to the target tumour cells. RI-p16MIS-4R: GPG-rhlvvltdlf-GP-RRRR. (lower case letters;D-amino acids). Scale bars, 10 μm. Figure 4: Design of CPP-fusion anti-tumour peptide restoring p16INK4a function. ( a ) RT–PCR analysis of the p16 tumour suppressor gene and its target gene expression in the indicated primary tumour cells. HeLa and NHDF; positive control. Arrowheads depict the PCR product of each gene. ( b ) Anti-tumour peptide design. Capital letters; L -amino acid. Lower case letters; D -amino acid. Each peptide was tagged with four arginines at its C-terminus to enhance solubility. ( c ) Specificity of the interaction of the retro-inverso-designed p16MIS peptide targeting p16, the Cdk4/CyclinD1complex. Real-time BIACORE sensorgrams of the interaction between the indicated peptide and the Cdk4/CyclinD1 protein complex, and the graph as a summary. Loaded peptide; 0.125, 0.25, 0.5, 1, 2 μM conc., respectively. RU; resonance unit, RU/KD; Relative Response/Molecular weight. D -p16MIS, the retro-inverso form of p16MIS showed maximum affinity to the target protein complex with the same doses. ( d ) Permeability of the CPP44- or CPP2-fusion chimeric p16MIS anti-tumour peptides to the target tumour cells. RI-p16MIS-4R: GPG-rhlvvltdlf-GP-RRRR. (lower case letters; D -amino acids). Scale bars, 10 μm. 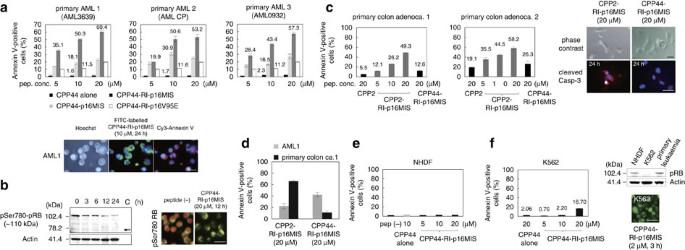Figure 5: Anti-tumour activity of tumour lineage-homing CPP44 or CPP2-fusion peptidein vitro. (a) Induction of apoptosis in three primary AML cell lines treated with CPP44-fusion p16 peptides. FACS analysis using Annexin V (upper panel); image of Annexin V-positive AML cells treated by CPP44-RI-p16MIS (lower panel). Means and s.d. of triplicates are shown. (b) Time-course-dependent decrease of phosphorylated serine 780 of pRB protein in AML cells treated with 20 μM CPP44-RI-p16MIS shown by immunoblotting (upper panel); loss of phospho-Ser780 pRB expression by imunofluorescence (lower panel). (c) FACS analysis using Annexin V for primary colon cancer cells treated with CPP2-RI-p16MIS. CPP44-RI-p16MIS was less effective on colon cancer cells. Means and s.d. of triplicates are shown. Primary colon adenocarcinoma cells incubated with CPP2-RI p16MIS were positive for cleaved caspase-3 (cy3-labelled). (d) Tumour lineage-specific effects of each anti-tumour peptide evaluated by FACS using Annexin V. The primary AML or primary colon adenocarcinoma cells were incubated with the indicated peptide and were analysed 24 h post-introduction. Means and s.d. of triplicates are shown. (e) The effect of CPP44-RI-p16MIS on non-neoplastic NHDF measured by FACS. Means and s.d. of triplicates are shown. (f) Weak apoptotic reaction on K562 cells by CPP44-RI-p16MIS. K562 lacked pRB protein expression, although peptide was efficiently incorporated. Means and s.d. of triplicates are shown. Scale bars (a,b,c,f), 10 μm. Full size image Figure 5: Anti-tumour activity of tumour lineage-homing CPP44 or CPP2-fusion peptide in vitro . ( a ) Induction of apoptosis in three primary AML cell lines treated with CPP44-fusion p16 peptides. FACS analysis using Annexin V (upper panel); image of Annexin V-positive AML cells treated by CPP44-RI-p16MIS (lower panel). Means and s.d. of triplicates are shown. ( b ) Time-course-dependent decrease of phosphorylated serine 780 of pRB protein in AML cells treated with 20 μM CPP44-RI-p16MIS shown by immunoblotting (upper panel); loss of phospho-Ser780 pRB expression by imunofluorescence (lower panel). ( c ) FACS analysis using Annexin V for primary colon cancer cells treated with CPP2-RI-p16MIS. CPP44-RI-p16MIS was less effective on colon cancer cells. Means and s.d. of triplicates are shown. Primary colon adenocarcinoma cells incubated with CPP2-RI p16MIS were positive for cleaved caspase-3 (cy3-labelled). ( d ) Tumour lineage-specific effects of each anti-tumour peptide evaluated by FACS using Annexin V. The primary AML or primary colon adenocarcinoma cells were incubated with the indicated peptide and were analysed 24 h post-introduction. Means and s.d. of triplicates are shown. ( e ) The effect of CPP44-RI-p16MIS on non-neoplastic NHDF measured by FACS. Means and s.d. of triplicates are shown. ( f ) Weak apoptotic reaction on K562 cells by CPP44-RI-p16MIS. K562 lacked pRB protein expression, although peptide was efficiently incorporated. Means and s.d. of triplicates are shown. Scale bars ( a , b , c , f ), 10 μm. Full size image Potential applications of tumour lineage-homing CPPs Next, we investigated whether our in vitro findings were consistent in vivo . First, in vivo delivery of FITC-labelled CPP2 and CPP44 was examined in a mouse model of xenograft human tumour cells. For this purpose, human primary AML cells were orthotopically transplanted into the abdominal cavity of NOD-SCID mice to monitor intraperitoneal metastases. In this model, multiple metastases in the peritoneum and at the mesenteric lymph nodes were observed with massive bloody tumour ascites 14 days after intraperitoneal injection of 3×10 5 AML cells ( Fig. 6a ). The original AML cells and their GFP-derivatives were highly proliferative in vitro and in vivo ( Supplementary Fig. S5a ), and the mice implanted with 3×10 5 cells usually died of advanced tumours within 15 days. When FITC-labelled CPP44 was intraperitoneally injected, multiple micrometastases growing in the peritoneal cavity were detected under fluorescence stereomicroscopy by accumulation of the FITC-peptide at early tumour stages (10 days post-implantation) ( Fig. 6b ). In the model mice with advanced tumour dissemination at day 14, the fluorescent signal from neoplasms derived from FITC-labelled CPP44 was more intense than those from TAT or CPP2, and the metastatic foci were visualized underscoring the tumour uptake of CPP44 in vivo ( Fig. 6c ). Similarly, FITC-labelled CPP2 accumulated in intra-abdominal metastatic foci of primary human colon cancer cells in a xenograft mouse model. Transection of metastatic cancer tissue at the omentum showed CPP2 penetrating inside the tumour ( Fig. 6d ). Furthermore, the tumour mass and micrometastatic foci of hepatocellular carcinomas were also visualized on incorporation of FITC-CPP44; however, FITC-CPP44 did not efficiently accumulate in the colonic tumours in the same xenograft mouse models, as shown in Fig. 6d (also see Supplementary Fig. S5b ). As one of the major problems of in vivo CPP application is significant sequestration in the liver, we examined the in vivo distribution of the fluorescent CPP44 to various normal organs, including the liver, comparing it with those of tumour foci in AML cell-implanted mice. The uptake of intraperitoneally injected CPP by normal organs such as the liver, brain, lung, heart, kidneys, and intestines (partial intestinal fluorescence was due to residual feed) was faint in contrast to that of the tumour lesions ( Fig. 6e ). This preferential uptake of the CPP44 to target tumours was further confirmed with transections of pigmented organs including the heart, liver, spleen, and kidney in addition to non-pigmented organs ( Supplementary Fig. S5c ). Partial fluorescence at the renal pelvis is due to excretion process of the peptide in urinary system. A similar preferential uptake to tumour tissues was found with other CPPs; for example, CPP10 was efficiently incorporated into gastric adenocarcinoma in vivo without significant uptake by the stomach, spleen, or kidneys The incorporation of CPP10 was augmented in gastric cancer tissues compared with colon tumour tissues, indicating that CPP10 may be more useful for targeting invasive foci of gastric cancers ( Supplementary Fig. S5d ). Consequently, each CPP was able to accumulate in tumour lesions in vivo according to its corresponding tumour lineage transducing ability, in sharp contrast to normal tissues. 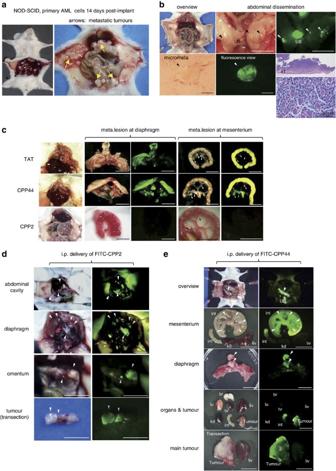Figure 6: Tumour imaging by lineage-homing CPPs in mouse tumour modelsin vivo. (a) Intra-abdominal development of primary AML cells (AML3639) in orthotopically transplanted NOD-SCID mouse. Accumulation of tumour ascites and multiple metastatic foci in the abdominal cavity (arrows). (b) Detection of micrometastatic tumours at the early stage by CPP44. FITC-labelled CPP44 (320 μg) was i.p. injected to mice at 10 days post-implantation of 3×105AML3639 cells. Mice were autopsied at 6 h post-injection of the FITC-peptide. Lowerview and hyperveiw of micrometastatic foci and corresponding lesions detected by the accumulation of FITC-CPP44. UB, urinary bladder; arrowheads, tumour lesions. Histology of the peritoneal tumour showed human myelogenous leukaemic cells. (c) Penetration of FITC-labelled TAT, CPP44, and CPP2 in the metastatic leukaemia lesionsin vivo. 14 days after implantation of 3×105tumour cells, 320 μg of each peptide was administrated intraperitoneally to the mice, which were autopsied 6 h post-injection. (d)In vivouptake of FITC-labelled CPP2 at metastatic foci in NOD-SCID mice implanted with human primary colon adenocarcinoma cells. Multiple intra-abdominal metastases depicted in FITC-labelled CPP2 (320 μg per mouse, i.p.). Scale bar, 10 mm. Arrowheads, tumour lesions. (e)In vivodistribution of CPP44 in AML cell-xenograft mice (14 days post-implantation). Fluorescent signals derived from accumulation of FITC-labelled CPP44 to target tumour tissues in comparison with non-neoplastic organs. UB, urinary bladder; int, small intestine; kd, kidney; liv, liver; br, brain; lu, lung; hr, heart. Scale bars are (b,c,d,e), 10 mm, except bottom panels of b 200 μm. Figure 6: Tumour imaging by lineage-homing CPPs in mouse tumour models in vivo . ( a ) Intra-abdominal development of primary AML cells (AML3639) in orthotopically transplanted NOD-SCID mouse. Accumulation of tumour ascites and multiple metastatic foci in the abdominal cavity (arrows). ( b ) Detection of micrometastatic tumours at the early stage by CPP44. FITC-labelled CPP44 (320 μg) was i.p. injected to mice at 10 days post-implantation of 3×10 5 AML3639 cells. Mice were autopsied at 6 h post-injection of the FITC-peptide. Lowerview and hyperveiw of micrometastatic foci and corresponding lesions detected by the accumulation of FITC-CPP44. UB, urinary bladder; arrowheads, tumour lesions. Histology of the peritoneal tumour showed human myelogenous leukaemic cells. ( c ) Penetration of FITC-labelled TAT, CPP44, and CPP2 in the metastatic leukaemia lesions in vivo . 14 days after implantation of 3×10 5 tumour cells, 320 μg of each peptide was administrated intraperitoneally to the mice, which were autopsied 6 h post-injection. ( d ) In vivo uptake of FITC-labelled CPP2 at metastatic foci in NOD-SCID mice implanted with human primary colon adenocarcinoma cells. Multiple intra-abdominal metastases depicted in FITC-labelled CPP2 (320 μg per mouse, i.p.). Scale bar, 10 mm. Arrowheads, tumour lesions. ( e ) In vivo distribution of CPP44 in AML cell-xenograft mice (14 days post-implantation). Fluorescent signals derived from accumulation of FITC-labelled CPP44 to target tumour tissues in comparison with non-neoplastic organs. UB, urinary bladder; int, small intestine; kd, kidney; liv, liver; br, brain; lu, lung; hr, heart. Scale bars are ( b , c , d , e ), 10 mm, except bottom panels of b 200 μm. Full size image On the basis of these results, we evaluated the potential therapeutic utility of these CPPs in vivo . CPP44-RI-p16MIS was administrated intraperitoneally 4 times every 12 h to mice with implanted human AML cells (AML3639) to examine anti-tumour activity. At day 14 post-implantation, most of the mice in the control group (vehicle only) had succumbed to aggressive tumours with full bloody tumour ascites, whereas the mice treated with CPP44-RI-p16MIS showed no significant accumulation of tumour ascites at this time point ( Supplementary Fig. S6a ). Survival analysis revealed that the CPP44-RI-p16MIS-treated mice showed statistically significant enhanced survival (mean survival, m.s., 20.8 days), compared with vehicle-treated mice (m.s., 14.3 days) ( P =0.0006<0.001) or mice treated with control peptides, including both CPP44-RI-p16V95E (m.s., 15.8 days) and TAT-RI-p16 (m.s., 16.3 days) ( P =0.0006<0.001, respectively), owing to substantial reductions in tumour growth and in ascites ( Fig. 7a ). Mann–Whitney tests indicated statistical significance with a P -value=0.0032 (both vehicle versus CPP44-RI-p16MIS, and CPP44-RI-p16V95E versus CPP44-RI-p16MIS) (data not shown). 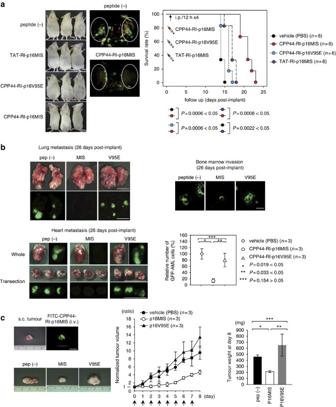Figure 7:In vivotherapeutic effect of tumour lineage-homing CPP-fusion p16 peptide. (a) Survival analysis byin vivodelivery of CPP44-RI-p16MIS peptide to peritoneally leukaemia-transplanted model mice. Appearance of the tumour-bearing mice with abdominal swelling caused by tumour ascites in the peptide-free group (PBS only), TAT-fusion p16 peptide-treated group, and the V95E control peptide-treated group showed abdominal swelling in contrast to mice treated with CPP44-RI-p16MIS (left). Macroscopic differences in intra-abdominal development of tumours in GFP-expressing AML3639 cell-implanted mice with or without CPP44-RI-p16MIS treatment. Dotted circles represent peritoneal metastases. Kaplan–Meier curves for overall survival of animals treated four times with the indicated peptide (i.p. injection of the peptide; 320 μg per injection per 12 h, repeated 4 times). (b) Development of multiple metastatic foci in NOD-SCID mice intravenously administrated with GFP-expressing human AML cells (AML3639). The mouse group without peptide treatment (pep(−)), that treated with CPP44-RI-p16MIS, and that with CPP44-RI-p16V95E (control peptide) were examined by autopsy at 26 days post-administration. Fluorescent foci of the lungs and hearts corresponded to the metastases of the GFP-AML cells in visible light fields (left). Bone marrow involvement of the engrafted AML cells in each mouse group is shown in fluorescent cell images (right upper panel). The comparative percentage of leukaemic cell involved in bone marrow among the three groups is shown in the graph (t-test). Means and s.d. of triplicates are shown. (c) Growth retardation of subcutaneously xenografted AML tumours in mice by treatment with anti-tumour peptide. Mice bearing subcutaneous AML3639 xenografts were started to be treated with vehicle (PBS-) alone, CPP44-RI-p16MIS, or CPP44-RI-p16V95E, when tumour volumes were ~100 mm3(that is, day 0). Tumour-bearing mice in each group were subjected to intravenous administration of the peptide once per day, for 8 days in a row. Gross appearance of the representative tumour of each group excised at day 8 (left panel). Tumour volumes were daily measured from day 0 to day 8. The volumes were normalized to initial tumour volumes on day 0 (initial volume as 1.0) as shown in the graph (middle)28. Statistical significances of tumour volumes and weights were evaluated by Student'st-tests. Vehicle (n=3, m.v. ratio 11.4 on day 8) versus CPP44-RI-p16MIS (n=3, m.v. ratio 4.65 on day 8);P=0.024<0.05, CPP44-RI-p16V95E (n=3, m.v. ratio 13.42 on day 8) versus CPP44-RI-p16MIS;P=0.017<0.05, vehicle versus CPP44-RI-p16V95E;P=0.36 >0.05,t-tests. Arrows indicate i.v. injection of the peptides or vehicle. Final tumour weights excised on day 8 in each group were also shown in the graph (right). Vehicle (n=3, m.w. 460 mg) versus CPP44-RI-p16MIS (n=3, m.w. 214 mg); *P=0.007<0.05, CPP44-RI-p16V95E (n=3, m.w. 652 mg) versus CPP44-RI-p16MIS; **P=0.047<0.05, vehicle versus CPP44-RI-p16V95E; ***P=0.194>0.05,t-tests. Means and s.d. of triplicates are shown. Scale bars on macroscopic images of the organs (b,c), 10 mm. Scale bar on cellular image (b), 10 μm. m.w., mean tumour weight. Figure 7: In vivo therapeutic effect of tumour lineage-homing CPP-fusion p16 peptide. ( a ) Survival analysis by in vivo delivery of CPP44-RI-p16MIS peptide to peritoneally leukaemia-transplanted model mice. Appearance of the tumour-bearing mice with abdominal swelling caused by tumour ascites in the peptide-free group (PBS only), TAT-fusion p16 peptide-treated group, and the V95E control peptide-treated group showed abdominal swelling in contrast to mice treated with CPP44-RI-p16MIS (left). Macroscopic differences in intra-abdominal development of tumours in GFP-expressing AML3639 cell-implanted mice with or without CPP44-RI-p16MIS treatment. Dotted circles represent peritoneal metastases. Kaplan–Meier curves for overall survival of animals treated four times with the indicated peptide (i.p. injection of the peptide; 320 μg per injection per 12 h, repeated 4 times). ( b ) Development of multiple metastatic foci in NOD-SCID mice intravenously administrated with GFP-expressing human AML cells (AML3639). The mouse group without peptide treatment (pep(−)), that treated with CPP44-RI-p16MIS, and that with CPP44-RI-p16V95E (control peptide) were examined by autopsy at 26 days post-administration. Fluorescent foci of the lungs and hearts corresponded to the metastases of the GFP-AML cells in visible light fields (left). Bone marrow involvement of the engrafted AML cells in each mouse group is shown in fluorescent cell images (right upper panel). The comparative percentage of leukaemic cell involved in bone marrow among the three groups is shown in the graph ( t -test). Means and s.d. of triplicates are shown. ( c ) Growth retardation of subcutaneously xenografted AML tumours in mice by treatment with anti-tumour peptide. Mice bearing subcutaneous AML3639 xenografts were started to be treated with vehicle (PBS-) alone, CPP44-RI-p16MIS, or CPP44-RI-p16V95E, when tumour volumes were ~100 mm 3 (that is, day 0). Tumour-bearing mice in each group were subjected to intravenous administration of the peptide once per day, for 8 days in a row. Gross appearance of the representative tumour of each group excised at day 8 (left panel). Tumour volumes were daily measured from day 0 to day 8. The volumes were normalized to initial tumour volumes on day 0 (initial volume as 1.0) as shown in the graph (middle) [28] . Statistical significances of tumour volumes and weights were evaluated by Student's t -tests. Vehicle ( n =3, m.v. ratio 11.4 on day 8) versus CPP44-RI-p16MIS ( n =3, m.v. ratio 4.65 on day 8); P =0.024<0.05, CPP44-RI-p16V95E ( n =3, m.v. ratio 13.42 on day 8) versus CPP44-RI-p16MIS; P =0.017<0.05, vehicle versus CPP44-RI-p16V95E; P =0.36 >0.05, t -tests. Arrows indicate i.v. injection of the peptides or vehicle. Final tumour weights excised on day 8 in each group were also shown in the graph (right). Vehicle ( n =3, m.w. 460 mg) versus CPP44-RI-p16MIS ( n =3, m.w. 214 mg); * P =0.007<0.05, CPP44-RI-p16V95E ( n =3, m.w. 652 mg) versus CPP44-RI-p16MIS; ** P =0.047<0.05, vehicle versus CPP44-RI-p16V95E; *** P =0.194>0.05, t -tests. Means and s.d. of triplicates are shown. Scale bars on macroscopic images of the organs ( b , c ), 10 mm. Scale bar on cellular image ( b ), 10 μm. m.w., mean tumour weight. Full size image We further examined the anti-tumour activity of the peptide in mice with intravenously (i.v.) administrated human AML cells. One week after injection of GFP-expressing AML cells in the tail vein, the mice were treated with CPP44-RI-p16MIS, CPP44-p16V95E, or with vehicle only (PBS-), respectively. The course of the peptide treatment was repeated a total of three times with a 5-day interval between each course, then mice were autopsied at 26 days post-implantation to examine leukaemic cell expansion in vivo . As a result, the group treated with CPP44-RI-p16MIS showed no metastasis to the lung and heart, whereas both of the no-peptide group and the V95E-treated group developed multiple metastases of the lung and massive invasion of the heart ( Fig. 7b ). Histologically, the mice of the control groups (vehicle and V95E) showed multiple micrometastases adjacent to the small blood vessels in the lungs, and these were positive for the myeloid cell marker, CD33 ( Supplementary Fig. S6b ). In one of the V95E peptide-treated mice, liver and spleen metastases were also observed ( Supplementary Fig. S6c ). An increased number of GFP-expressing leukaemic cells were detected on cytosmear specimens of freshly isolated bone marrow cells from the mice in the control groups (vehicle only; that is, peptide (−), and V95E groups), whereas the number of invasive cells was approximately one-seventh of the controls in the MIS-treated mice ( n =3; average number in the untreated group, 27.7 cells per 500 cells; 3.8/500 in the MIS-treated group; 21.8/500 in the V95E-treated group) ( Fig. 7b ; Supplementary Fig. S6d ). Consequently, the percentage of bone marrow involvement was relatively small, at 14% in the p16MIS-treated mice, and 79% in the V95E-treated mice that is similar to the base number in the untreated mice (standardized as 100%). The result was statistically significant (p16MIS versus vehicle, P =0.019<0.05; p16MIS versus p16V95E, P =0.033<0.05, t -tests) ( Fig. 7b ). The therapeutic effect of intravenously administrated CPP44-RI-p16MIS peptide were finally examined on subcutaneous xenograft AML tumour in mice. Examination by fluorescence stereoscopy revealed that the peptide was successfully absorbed to the target tumour by i.v. injection ( Fig. 7c ). Growth retardation of the tumours was observed in mice of the CPP44-RI-p16MIS-treated group in comparison with those in mice of peptide-untreated and the V95E-treated groups, which was demonstrated by a decrease in tumour size, volume and weight ( Supplementary Fig. S6e ), with statistical significances ( Fig. 7c ). To examine the in vivo toxicity of the anti-tumour peptide, CPP44-RI-p16MIS, serological analysis was performed for mice repeatedly treated with the anti-tumour peptide. Consequently, serologic tests revealed no significant abnormality in the peptide-treated mice in comparison with those without treatment. All values from both groups were within normal limits. ( Supplementary Fig. S6f ). CPPs have significant biomedical potential as noninvasive agents for molecular delivery via macropinocytosis and endocytosis [1] , [22] . The HIV-1-TAT peptide has been extensively used as the CPP molecule of choice in numerous studies. However, one of the most critical issues in molecular delivery systems for targeting cancer is tissue specificity for optimizing therapeutic efficiency. In the present study, novel CPPs were obtained by mRNA display technology, and the tumour lineage specificity of each newly synthesized CPP was discovered through functional screening. In this study, we found that only a single amino-acid substitution is needed to give rise to alternations in target cell selectivity in some cases ( Table 2 ; Fig. 1b,c ). The amino-acid sequences of these CPPs possess relatively few (typically <30%) positively charged amino acids such as lysine or arginine, in contrast to current CPPs such as TAT, SV40 NLS and polyarginine [23] . A protein database search revealed that these CPPs seem to encode artificial sequences as they have no significant identity to any recorded mammalian proteins, including previously reported CPP sequences. To investigate the mechanism of selective permeability of these novel CPPs, we selected CPP44, which displayed a high level of transduction in myelogenous leukaemias and hepatic tumours. With siRNA library screening, endogenous M160 (CD163L1; scavenger receptor cysteine-rich type I) expression seemed to be critical for CPP44 penetration ( Fig. 3d ). Its expression is abundant in myelogenous leukaemias and hepatic tumours, but not in normal human liver cells, fibroblasts, and low expression in other tumour lineages ( Fig. 3e ; Supplementary Fig. S2e ). Previous studies have suggested that CD163 (also known as M130) is exclusively expressed in monocyte/macrophage cell lineages, and CD163L1 (M160) also seems to be expressed in alveolar macrophages and monocyte-derived cell lines HL60, U937, and THP1 (refs 24 , 25 ). The family shares SRCR domains, like Ig domains or epidermal growth factor-like domains, which are thought to be involved in protein–protein interactions such as the binding and internalizing of hemoglobin–haptoglobin complexes. Although little is known about the biological role of M160 within other cells types, including malignant tumours, certain lineages of tumour cells may require its expression for promoting growth. Thus, it might be that a target molecule to each tumour-homing CPP exists, which is tumour lineage-dependently expressed, and may selectively facilitate the incorporation of the specific CPP. With regard to tumour-homing CPPs, it is important to restrict function to tumour tissues in vivo . Our in vivo analysis of intraperitoneally injected fluorescence-labelled CPP44, employing both metastatic leukaemic tumour and hepatic cancer-bearing mouse models, showed that the administrated peptide preferentially accumulated in metastatic tumour sites. Moreover, CPP44 was not significantly sequestered in the liver or in other normal organs such as the brain, lung, heart, intestine or the kidneys as shown ( Fig. 6e ; Supplementary Fig. S5b ). Similar results were observed for in vivo distribution of CPP2 and CPP10 ( Fig. 6d; Supplementary F S5d , respectively). An important technical issue in the present study is modulating the dosage of the tumour-homing peptides for future practical utilization. We used fluorescence-labelled CPPs as a tool for imaging metastatic tumours in a mouse model in this study, but, for example, radionuclide-labelled forms may minimize the dosage as well as use in a detection system. As an initial attempt at therapeutic application of a tumour-homing CPP, we generated the anti-tumour peptide, CPP44-RI-p16MIS, and applied it to AML-xenograft mouse models. Administration of the peptide resulted in prolonged survival of the treated mice and inhibition of tumour expansion in vivo . In a mouse model with intravenous administration of human GFP-expressing AML cells, metastases to the lung and heart rapidly occurred before bone marrow invasion due to the abundant blood flow. Consequently, these organs were massively occupied with tumour cells and the mice of the control groups were seriously weakened by 26 days post-implantation when the bone marrow still showed early stage invasion. However, mice treated with CPP44-fusion p16 peptide were still active at this time point, and an anti-tumour effect of the peptide was confirmed. This inhibitory effect was also corroborated by a subcutaneous tumour mouse model, using intravenously administrated peptide. As shown in the graph, the average time for tumour volumes to reach four times the starting volume was approximately 48 h in peptide-untreated (vehicle only) group, 74 h in CPP44-RI-p16V95E-treated group, and 170 h in CPP44-RI-p16MIS-treated group, which showed significantly longer in mice treated with the p16MIS peptide. Daily treatment of the mice by the CPP44-p16 functional peptide resulted in an ~50% reduction of tumour volume and weight at end point in comparison with those in control groups. Histological examination revealed tumours treated with CPP44-RI-p16MIS seemed to involve more prominent multiple degenerated lesions inside than the peptide-untreated tumours ( Supplementary Fig. S6e ). Thus, the CPP44-p16 peptide showed in vivo anti-tumour function to some extent, even though it did not completely eradicate the tumours. Meanwhile, serological examination revealed there was no pathological damage to non-neoplastic tissues in vivo after repeated administration of the peptide ( Supplementary Fig. S6f ). Taken together, representative CPPs such as CPP2 and CPP44 can home into tumour cells and tissues according to their lineage specificities in vitro and in vivo . These CPPs noninvasively target their corresponding tumours minimizing transduction into normal tissues. In conclusion, the tumour lineage-homing CPPs, generated by mRNA display technology, are potentially useful tools for developing peptide-based molecular delivery systems in cancer biology in addition to an array of other fields. Peptide synthesis and sequence information All peptides were purified to HCl form by reverse-phase high-performance liquid chromatography (HPLC), to >95% purity for both in vitro and in vivo applications (Sigma-Aldrich, Japan). Peptide identities were confirmed by mass spectrometry. For synthesis of p16 MIS, the 10 sequential amino-acid residues 'FLDTLVVLHR,' identified as the MIS of p16 by Fahraeus et al . [19] , was considered the core of the peptide with respect to restoring p16 function. FITC was conjugated at the NH 2 -terminus of a peptide via a 6-aminohexanoic acid linker (Ahx). Secondary structural predictions of CPP44 derivatives were obtained by sequence analysis of each particular peptide using PROTANAS for Win (Kyoritsu Shuppan, Japan) and Chem3D Pro 8.0 (HULINKS, Tokyo, Japan) software. Tumour cell lines and primary tumour cells Tumour cell lines were purchased from American Type Culture Collection, or supplied by Hayashibara Biochemical Laboratories (Okayama, Japan). FL-18 was provided by Dr H. Ohno (Takeda Hospital) and HCC lines were supplied by Dr H. Yano (Kurume University). Primary colonic cancer cells were freshly isolated from surgically excised primary tumour tissues from two patients with colon adenocarcinoma. Similarly, primary AML cells were isolated from bone marrow-biopsied tissues from two patients at initial diagnosis at Okayama University Hospital, and the cells in one case were obtained from CelProgen by Material Transfer Agreement. Following the second-to-third subcultures, the resulting primary cells were utilized for the in vitro and in vivo assays. The studies using the patient-derived primary cells and healthy volunteers' PBMCs were approved by the research ethics committees of Okayama University and the Aichi Cancer Center. Informed consent was also obtained from each patient for use of the primary tumour cells. Fluorescence cellular imaging Uptake and intracellular localization of FITC-labelled CPPs and CPP-fusion p16 peptides were visualized in live cells by an inverted fluorescence microscope. For the first cell-penetration assay, using the synthesized CPPs to established tumour cell lines, fluorescent images were obtained from cells treated with 10 μM of peptide for 6 h. Images for in vitro primary cell-penetration assays were obtained from cells treated with 10 μM of the fluorescent peptides for 3-h incubations. For the drug-mediated inhibitory assay, cells were incubated in 2 μM CPPs for 1 h against the peptide-uptake using EIPA, DI or CPZ, and knockdown assays by siRNA. Before taking fluorescence images of incorporated CPPs in vivo , mice were autopsied following 6 h treatments with intraperitoneally injected peptides. They were examined by zoom stereo fluorescence microscopy immediately after autopsy. Quantitative fluorescent image analysis Fluorescent intensities of the microscopic images obtained from the tumour lines, incorporating FITC-labelled tumour-homing CPPs, were measured with MetaMorph software Version 6 (Olympus, Japan). Living cells exhibiting normal nuclear morphology were considered with respect to acquisition of fluorescence intensity per cell; furthermore, analysis was performed utilizing the entire soma of individual cells as the region of interest. The fluorescence intensity of 20 cells was counted; three sets of experiments were conducted. Background fluorescence intensity was subtracted from all experiments. Flow cytometric analysis Cytocidal assays were performed using the Cy3-Annexin V staining kit on peptide-treated tumour cells. In total 10,000 cells were examined in each sample (FACScan, Becton Dickinson, USA). Cell cycle analysis was also performed by FACScan, using propidium iodide staining [20] , [21] . Imunoblotting The extracts of peptide-treated cells were separated by SDS–PAGE using 4–12% bis-Tris gradient or 3–8% Tris-acetate gels. Blotted membranes were sequentially probed with the anti-phospho-Ser780 pRB 1:300 (Cell Signaling Technology), anti-total pRB 1:300 (Cell Signaling Technology), anti-M160 rabbit polyclonal antibodies 1:500 (Sigma-Aldrich), or anti-actin monoclonal antibody 1:20,000 (Chemicon) [20] . RT–PCR Two μg of total RNA were extracted from tumour cells and converted to complementary DNA using an oligo(dT) primer and reverse transcriptase for performing PCR. The sense/antisense primer sequences for p16 INK4a , Cdk4 , Cdk6, CyclinD1 , RB and GAPDH were as described previously [20] , [26] . p16INK4a: sense primer; 5′-ATGGAGCCGGCGGCGGGGAG-3′, antisense primer; 5′-TCAATCGGGGATGTCTGAGG-3′ Cdk4: sense primer; 5′-TGACAAGTGGTGGAACAGTC-3′, antisense primer; 5′-TAAGAGTGCTGCAGAGCTCG-3′ Cdk6: sense primer; 5′-TCTTGCTCCAGTCCAGCTAC-3′, antisense primer; 5′-AGCAATCCTCCACAGCTCTG-3′ CyclinD1: sense primer; 5′-GAGGAACAGAAGTGCGAGGA-3′, antisense primer; 5′-TCTGGAGAGGAAGCGTGTGA-3′ RB: sense primer; 5′-CTTGCATGGCTCTCAGAT-3′, antisense primer; 5′-AGATTAAGAGGACAAGCA-3′ GAPDH: sense primer; 5′-GGTGAAGGTCGGAGTCAACGGA-3′, antisense primer; 5′-GAGGGATCTCGCTCCTGGAAGA-3′ Primers for M160 (α-form of CD163L1) : sense 5′-AGATGCTGCTGTCATCAGAACCTT-3′, antisense 5′-TTTGCACACGACAGTTGAGGCAGTA-3′. siRNA library screening and knockdown assay To identify the responsible gene for CPP44 incorporation, a total of 1,905 siRNAs against the receptor genes were screened by lipofection to primary AML cells (AML3639) first, using an siRNA library for human receptor genes (siPerfect Library; Sigma-Aldrich). The FITC-labelled CPP44 uptake to the target cells (final conc. 2 μM, incubated for 3 h) was evaluated with fluorescence microscopy 48 h after transfection of 50 nM of siRNA. The effect of M160 mRNA knockdown on peptide uptake was examined and confirmed by independent introduction of 50 nM siRNA against M160 with different sequences (ON-TARGET plus SMART Pool siRNA (Thermo Scientific, USA) and Validated MISSION si (Sigma-Aldrich, USA)). An equal amount of ON-TARGET plus Non-Targeting Pool (Thermo Scientific, USA) was used as a negative control siRNA. Surface plasmon resonance analysis for designed p16 peptides Binding kinetics between the p16MIS peptides and their target, the Cdk4/CyclinD1 complex, were measured by a surface plasmon resonance assay utilizing a Biacore T200 biosensor system. A mixture of recombinant Cdk4 and CyclinD1 protein at equal molar ratios (Abcam) was immobilized on CM5 sensor chips at a concentration of 50 μg ml −1 in 10 mM phosphate buffer, pH 6, using the coupling kit supplied by the manufacturer. Relative Response/Molecular weight was calculated from each peptide/target complex interaction following the T200 biosensor program. Peptides used for surface plasmon resonance assay were: L -16 (p16MIS; FLDTLVVLHR), D -p16 (retro-inverso form of p16MIS; rhlvvltdlf), D -p16V95K (rhlvkltdlf), D -p16V95E (rhlveltdlf), and D -p16 scram (scrambled form of D -p16; rvdtlhvfl). Capital letters, L -amino acids; lower case letters, D -amino acids. Mouse tumour models and in vivo anti-tumour peptide delivery A total of 3.0.×10 5 cells of human AML cells (AML3639, isolated from the patient) were transplanted into the peritoneal cavity of a 7-week-old NOD-SCID mouse by direct injection. For a colon cancer model, 1×10 6 of primary colon adenocarcinoma cells (second passage) were implanted in the same manner. Survival was measured in six CPP44-RI-p16MIS peptide-treated mice compared against the same number of vehicle-treated or control CPP44-RI-p16V95E-treated mice. 320 μg of the peptide dissolved in PBS was intraperitoneally injected per mouse for a total of four times, once every 12 h. For intravenous delivery of the AML cells, 2.0×10 6 of AML3639 cells were administrated in the tail veins of NOD-SCID mice. A week after the injections, mice were treated with the same dose of the intraperitoneally injected peptide or with vehicle (PBS) once per day for 3 days (320 μg per mouse per day) as a course, and the course of treatment was repeated a total of three times with 5-day intervals. Twenty-six days after initial administration of the tumour cells, all mice were autopsied and their organs examined by fluorescence stereomicroscopy. At the same time, bone marrow cells were freshly collected from the murine femoral bones of each group at autopsy after removal of red blood cells by treatment with Tris-buffered ammonium chloride. Bone marrow involvement of the GFP-expressing AML cells in the intravenously xenografted mice were evaluated by preparing cytosmears. The number of GFP-expressing cells, out of a total of 500 cells, was counted on the specimens from a mouse belonging to each group (non-treated, vehicle only, CPP44-RI-p16MIS-treated, CPP44-RI-p16V95E-treated). Then, the relative percentages of bone marrow invasion were calculated based on the number of invasive cells in the MIS-treated group against that of the non-treated group, and the V95E-treated group against the non-treated group. For subcutaneous xenograft models, 2.0×10 6 of AML3639 cells were subcutaneously injected to the 7-week-old NOD-SCID mice. When volume of the xenograft tumours reached ~100 mm 3 , CPP44-RI-p16MIS, CPP44-RI-p16V95E, or vehicle (PBS-) alone, was intravenously administrated to mice once per day for 8 days from day 0 to day 7, that is, totally 8 times in a row (600 μg i.v. per mouse per day, each group; n =3 mice). Tumour volumes in each group were calculated everyday [27] as (length×width) 2 ×0.5 mm 3 . On day 8, tumours of each group were surgically excised and their weights were measured for comparison in addition to tumour sizes. Uptake of CPP44-RI-p16MIS peptide was confirmed by excised subcutaneous xenograft tumour (~100 mm 3 as a volume) 6 hours after intravenous administration of the FITC-labelled peptide (600 μg i.v.). For the serological analysis to examine the toxicity of the CPP44-RI-p16MIS peptide in vivo , the peptide was intraperitoneally administrated to healthy NOD-SCID mice a total of four times with a 7 day-interval between each administration. Serum samples were collected from these 7 days after the final injection and were measured. The animal studies in the present work were approved by the Aichi Cancer Center on Animal Research. All mouse procedures and euthanasia, including cell transplantations and peptide injections, were done painlessly or under anaesthesia, within the strict guidelines of the Experimental Animal Committees of Aichi Cancer Center Research Institute. Statistical analysis Statistical significance was calculated using the statistics software package StatView (SAS, USA). Survival curves were generated by the Kaplan–Meier method. P <0.05 was considered statistically significant. The samples with bone marrow invasion of GFP-expressing AML cells, tumour volumes and weights were statistically analysed by Student's, t -test. P <0.05 was considered statistically significant. How to cite this article: Kondo, E. et al . Tumour lineage-homing cell-penetrating peptides as anticancer molecular delivery systems. Nat. Commun. 3:951 doi: 10.1038/ncomms1952 (2012).